Templated three-dimensional growth of quasicrystalline lead Quasicrystals, materials with aperiodic long-range order, have been found in intermetallics, soft materials such as colloids and supermolecules, and also in two-dimensional monolayer films. Here we present the first example of three-dimensional growth of a single-element quasicrystalline film. Using a hitherto unexplored template, the icosahedral Ag-In-Yb quasicrystal, and various experimental techniques combined with theoretical calculations of adsorption energies, we find that lead atoms deposited on the surface occupy the positions of atoms in the rhombic triacontahedral cluster, the building block of the substrate, and thus grow in layers with different heights and adsorption energies. We show that the adlayer–adlayer interaction is crucial for stabilizing this epitaxial quasicrystalline structure. The finding opens an avenue for further investigation of the impact of the aperiodic atomic order over periodic order on the physical and chemical properties of materials. Since their discovery [1] , quasicrystalline phases have been found in >100 intermetallic compounds, liquid crystals [2] , polymers [3] , colloids [4] and perovskite thin films [5] , and are recognized as universal phases of matter. A very important breakthrough was the discovery of stable intermetallic phases [6] , which enabled detailed experimental studies, including the determination of accurate atomic structures of quasicrystals and investigation of quasicrystalline surfaces and overlayers (ref. 7 and references therein). A universal pseudogap in the electronic density of states near the Fermi energy is characteristic of quasicrystals and related compounds [8] , and semiconducting electronic transport has been reported for many systems [9] . This unique electronic structure in turn affects physical and chemical properties of quasicrystal surfaces, resulting in unexpected surface properties such as non-stickiness and low friction [10] , [11] . Because of their unusual structure and rotational symmetry, quasicrystals provide unique templates for the exploration of new epitaxial phenomena. Several interesting results have been observed in adsorption on surfaces of the Al-based quasicrystals (ref. 7 and references therein), which include pseudomorphic monolayers of Bi [12] , [13] , Sb [12] , Pb [14] , [15] and Sn [16] , quasiperiodically modulated multilayer structures of Cu [17] , [18] and Co [19] , fivefold twinned islands with magic heights influenced by quantum size effects [20] and a non-fcc structure of Ag [21] . In this study, we demonstrate the formation of a novel form of quasicrystalline structure, which is formed by a single element grown on a template. Using the fivefold surface of the icosahedral ( i -) Ag-In-Yb quasicrystal as a substrate, we have succeeded in growing a quasicrystalline film of a single element where the adatoms occupy multiple sites at different levels, which correspond to the completion of the rhombic triacontahedral (RTH) bulk clusters truncated by the surface. This finding adds to previous observations of modulated multilayers and quasicrystalline monolayers observed on the common Al-based quasicrystals. Combining the experimental results using scanning tunnelling microscopy (STM), low-energy electron diffraction (LEED) and x-ray photoemission spectroscopy (XPS) with density functional theory (DFT) calculations for adsorption energies, we have determined the structure of the Pb film. The Pb atoms occupy the position of atoms in the RTH cluster, the building block of the Ag-In-Yb quasicrystal, and thus mirror the atomic positions in the truncated half cluster of the bulk. As a result of this, the structure of the film can be characterized by layers of atoms with different heights above the substrate. The structure of each layer can be deduced from the substrate structure. As such, each layer is geometrically distinct from the layer below, leading to the film as a whole displaying quasicrystalline order in three dimensions. Thus, this system constitutes the simplest possible quasicrystal. Substrate structure The i -Ag-In-Yb quasicrystal is isostructural to the unique binary i -Cd-Yb phase [22] , where Cd is replaced by Ag and In. The atomic structure of this system has been solved without ambiguity [23] . The basic building block of this system is the RTH cluster, which consists of five successive atomic shells [23] . Details about the structure and the thin-film preparation process is given in Methods. The substrate surface can be prepared with wide flat terraces ( Fig. 1a ). The terraces are formed preferentially at bulk planes, which are dense, Yb rich and intersect the cluster centres [24] . STM images taken at negative sample bias voltage are characterized by protrusions located at the vertices of a Penrose P1 tiling with an edge length of about 24±1 Å (ref. 24 ). The P1 tiling consists of four different tiles: pentagons, stars, rhombi and boats [25] . The pentagons are of two different orientations, rotated at 36° to each other. These are marked in Fig. 1a . 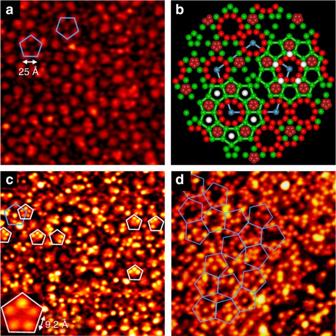Figure 1: Initial Pb adsorption sites. (a,c,d) STM images (300 Å × 300 Å) of a terrace of the fivefoldi-Ag-In-Yb surface (a, clean surface;c, after deposition of Pb for 5 min;d, 15 min). The substrate pentagonal features and Pb pentagons are marked by blue and white pentagons, respectively, inaandc. A patch of a Penrose P1 tiling is overlaid ind. (b) Atomic structure of a bulk-terminated surface ofi-Ag-In-Yb deduced from the structure ofi-Cd-Yb. The vertices of pentagonal unit are uniquely decorated by Ag/In rings (red) surrounded by Yb pentagons (green). Dark red spheres represent Ag/In atoms at 0.4 Å below the top layer and blue spheres the centre of RTH units. White spheres forming small and large pentagons mark adsorption sites for Pb atoms in the first and second layers. Figure 1: Initial Pb adsorption sites. ( a , c , d ) STM images (300 Å × 300 Å) of a terrace of the fivefold i -Ag-In-Yb surface ( a , clean surface; c , after deposition of Pb for 5 min; d , 15 min). The substrate pentagonal features and Pb pentagons are marked by blue and white pentagons, respectively, in a and c . A patch of a Penrose P1 tiling is overlaid in d . ( b ) Atomic structure of a bulk-terminated surface of i -Ag-In-Yb deduced from the structure of i -Cd-Yb. The vertices of pentagonal unit are uniquely decorated by Ag/In rings (red) surrounded by Yb pentagons (green). Dark red spheres represent Ag/In atoms at 0.4 Å below the top layer and blue spheres the centre of RTH units. White spheres forming small and large pentagons mark adsorption sites for Pb atoms in the first and second layers. Full size image The protrusions observed in STM are related to the cross-section of the Cd icosidodecahedral shell of the RTH cluster. To explain this, we present in Fig. 1b the atomic structure of surface-terminating bulk layers deduced from the ideal bulk model of i -Cd-Yb [23] . The icosidodecahedral shells of the RTH cluster form decagons at the surface (red rings in the figure), which are centred at the vertices of a P1 tiling of 25.3 Å edge length. According to the structure of the Ag-In-Yb approximant [26] , the icosidodecahedral shell is mostly occupied by In (see below for further discussion of the occupation probability of Ag and In). We will, therefore, refer to the decagon as the In decagon. The In decagon at each vertex of the P1 tiling is surrounded by ten Yb pentagons, which belong to different RTH units or to the glue atoms between the RTH clusters. In STM, large protrusions are observed at the positions of In decagons at negative bias, whereas the Yb pentagons are resolved at positive bias [24] . STM of Pb film Figure 1c shows an STM image after 5 min deposition of Pb, where the area covered by Pb atoms is about 10–20% of the total substrate area (about 2 × 10 −3 atoms per Å 2 ). At this low coverage, both the substrate structure and the deposited Pb atoms are resolved, and thus it is possible to identify the adsorption sites. The brighter dot-like motifs in the image correspond to individual Pb atoms, which are at a height of ~1.1±0.1 Å above the substrate. The Pb atoms form pentagons of 9.2±0.5 Å edge length (marked in Fig. 1c ). At this coverage, most pentagons are incomplete, and isolated Pb atoms are also observed. At increasing coverages, complete pentagons evolve. The Pb pentagons are observed on the top of the protrusions. They exhibit only one orientation, which is identical to one of the pentagonal units of the substrate. From the location with respect to the substrate, and the size and orientation of the Pb pentagons, an adsorption site is identified between the In and Yb rings. These sites are marked by five spheres forming a small white pentagon in Fig. 1b . On further deposition (15 min), a network of Pb pentagons is obtained as shown in Fig. 1d . The structure of the network can be mapped with a P1 tiling of edge length of ~25 Å, with the vertices located at the centres of the Pb pentagons. Such a tiling is expected from the substrate structure if Pb atoms occupy the selected adsorption sites mentioned above. The density of adatoms at this coverage deduced from STM images of different terraces varies from 4 × 10 −3 to 7 × 10 −3 atoms per Å 2 , which is less than the atomic density of the topmost substrate layer (3 × 10 −2 to 5 × 10 −2 atoms per Å 2 ), but in the same range as the density of the possible adsorption sites calculated from the substrate structure, suggesting that this coverage is close to saturation of these sites. Once the adsorption sites between the In and Yb rings are saturated, Pb atoms adsorb on top of the network of the Pb pentagons ( Fig. 2a ). These Pb atoms, which appear as red in the colour map, are at a height of 3.1±0.1 Å above the substrate and, thus, can be considered to be part of a second Pb layer above the network of Pb pentagons, which form the first layer. The Pb atoms in the second layer also form pentagons. These pentagons have an edge length of 13.8±1.5 Å, which is larger than the pentagons in the first layer by a factor of τ =1.618…, an irrational number characteristic of quasicrystalline order. They exhibit an identical orientation, rotated by 36° with respect to the pentagons in the first layer. This can be seen in Fig. 2a where pentagons of both layers are resolved. Both the size and orientation of the Pb pentagons suggest that Pb atoms in the second layer are adsorbed at the centre of alternating Yb pentagons surrounding the RTH cluster centres. These sites are marked by white spheres forming a large pentagon in Fig. 1b . 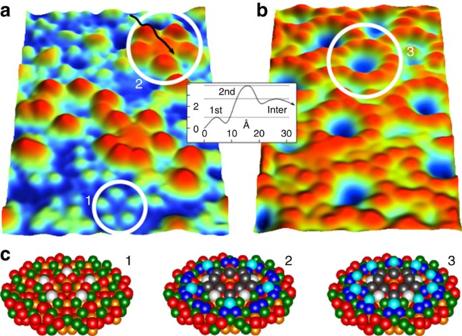Figure 2: Evolution of successive Pb layers. STM images (180 Å × 145 Å) of a terrace of the fivefoldi-Ag-In-Yb surface after deposition of Pb for 30 min (a) and 90 min (b). The inset is the height profile along a line indicated by an arrow, demonstrating the height of the first, second and intermediate layers. (c) Model structures corresponding to the white circles marked 1–3 inaandb, deduced from the calculations. Red spheres, Cd atoms; green, Yb; white, Pb in the first layer; blue, Pb in the second layer; grey, Pb in the intermediate layer. Figure 2: Evolution of successive Pb layers. STM images (180 Å × 145 Å) of a terrace of the fivefold i -Ag-In-Yb surface after deposition of Pb for 30 min ( a ) and 90 min ( b ). The inset is the height profile along a line indicated by an arrow, demonstrating the height of the first, second and intermediate layers. ( c ) Model structures corresponding to the white circles marked 1–3 in a and b , deduced from the calculations. Red spheres, Cd atoms; green, Yb; white, Pb in the first layer; blue, Pb in the second layer; grey, Pb in the intermediate layer. Full size image The Pb second-layer pentagon develops into a decagon with increasing coverage. The evolution to the decagon occurs when additional Pb atoms occupy the centre of the remaining Yb pentagons around the RTH cluster centre (refer to the model in Fig. 2c ). After 90 min deposition, a well-ordered network of Pb decagons is obtained ( Fig. 3a ), where the Pb decagons are located at the vertices of a P1 tiling as expected from the substrate structure. Some of the Pb decagons are occupied by a single Pb atom at the centre, which is at the same height as the decagon. The density of Pb atoms in the second layer is 7 × 10 −3 to 8 × 10 −3 atoms per Å 2 . This value is in agreement with the density of adsorption sites expected from the substrate structure (6 × 10 −3 to 8 × 10 −3 sites per Å 2 , that includes the centre of the RTH clusters). 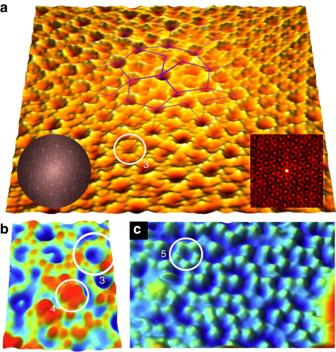Figure 3: Quasicrystalline Pb layers at different heights. (a) STM image (300 Å × 300 Å) of the fivefoldi-Ag-In-Yb surface after deposition of Pb for 90 min. Left inset: Fourier transform of the image. Right inset: a section of autocorrelation function of a 1,000 Å × 1,000 Å STM image (180 Å × 145 Å). A P1 tiling patch is overlaid, which is inflated byτwith respect to the tiling of the substrate or first layer. (b,c) STM images at the same coverage demonstrating the intermediate (b) and third layer (b: 300 Å × 300 Å;c: 270 Å × 150 Å) with quasicrystalline order. The white circles marked 3, 4 and 5 identify the second, intermediate and third layer features, respectively, discussed in the text. Figure 3: Quasicrystalline Pb layers at different heights. ( a ) STM image (300 Å × 300 Å) of the fivefold i -Ag-In-Yb surface after deposition of Pb for 90 min. Left inset: Fourier transform of the image. Right inset: a section of autocorrelation function of a 1,000 Å × 1,000 Å STM image (180 Å × 145 Å). A P1 tiling patch is overlaid, which is inflated by τ with respect to the tiling of the substrate or first layer. ( b , c ) STM images at the same coverage demonstrating the intermediate ( b ) and third layer ( b : 300 Å × 300 Å; c : 270 Å × 150 Å) with quasicrystalline order. The white circles marked 3, 4 and 5 identify the second, intermediate and third layer features, respectively, discussed in the text. Full size image A network of pentagons of two different orientations of edge length 15.8±1 Å is observed at 2.8±0.3 Å above the second layer and, thus, this network forms a third layer ( Fig. 3b ). The pentagons are inflated by τ with respect to the pentagons in the first layer and they form part of a P1 tiling. In addition to the first, second and third layers, Pb atoms at three other heights are also observed. Two of these additional layers are observed by STM below and above the second layer. We will refer to these layers as intermediate layers. The calculations discussed below reveal the existence of another layer in between the substrate and the first layer, and we will refer to this as an underlayer. This layer was not identified by STM, being underneath the first layer, but was detected by XPS. XPS probes the top few surface layers, whereas STM provides information on only the topmost layer. This technique also allows a determination of the growth mode and the amount of Pb adsorbed on the surface. At higher coverages, Pb develops three-dimensional, rotational epitaxial periodic islands with (111) surface orientation on top of the quasicrystalline film. Features of the intermediate layers are apparent in Figs 2a and 3b . A shallow broad feature identified in some of Pb decagons is measured at 1.0±0.1 Å below the second layer or ~1 Å above the first layer, as demonstrated by a height profile in Fig. 2 . These features develop simultaneously with the second layer Pb atoms (refer to the centre of the marked pentagon in Fig. 2a ). Similarly, a pentagon marked 4 in Fig. 3b is identified above the second layer and below the third layer. In addition to these pentagons, isolated Pb atoms are observed at the same height and, thus, these atoms constitute the intermediate layers. XPS and LEED To measure the growth curve by XPS, the intensity of core-level peaks of the substrate (In 3 d ) and film (Pb 4 f ) were measured as a function of Pb coverage, as plotted in Fig. 4a . A point of intersection of line segments with different gradients corresponds to a completion of a layer. Three inflection points are observed, indicating that three layers are successively formed. A comparison of STM and LEED results suggests that the first and second layers are completed at the first (11 min) and third (50 min) inflection points. The second inflection point (25 min) confirms the formation of an extra layer, the underlayer. As shown in the desorption curve in Fig. 4a (inset), the second layer starts to desorb at ~370 K (end of the first plateau in the graph) and the first layer at ~540 K. This further indicates that the two layers have non-identical binding energies, as expected from the growth of successive layers observed in the growth curve as well as in STM images. No inflection point corresponding to the other layers has been observed in the growth curve, possibly because they grow simultaneously with other layers or their density is too low to observe a break point. For the same reason, desorption temperatures of the other layers could not be determined from the desorption curve. 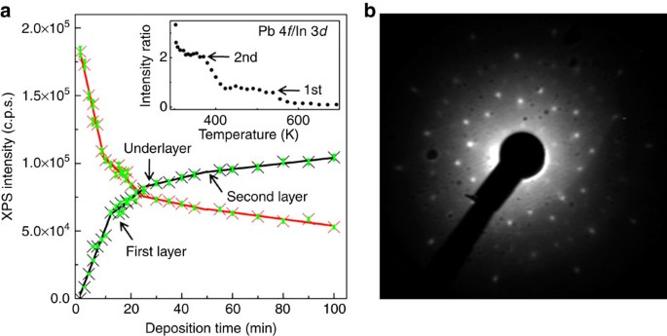Figure 4: Growth and stability, and long-range order of the Pb overlayer. (a) Variation of XPS intensity of the substrate (In 3d) and film (Pb 4f) as a function of deposition time, fitted with lines of different gradients. Error in intensity is shown by green bars. Inset: the ratio of Pb 4fand In 3dintensity after annealing the Pb-covered surface at different temperatures. The intensity corresponding to the first, second and underlayers is marked by arrows. (b) LEED pattern after formation of the second layer Pb taken using MCP-LEED optics (beam energy 24 eV). Figure 4: Growth and stability, and long-range order of the Pb overlayer. ( a ) Variation of XPS intensity of the substrate (In 3 d ) and film (Pb 4 f ) as a function of deposition time, fitted with lines of different gradients. Error in intensity is shown by green bars. Inset: the ratio of Pb 4 f and In 3 d intensity after annealing the Pb-covered surface at different temperatures. The intensity corresponding to the first, second and underlayers is marked by arrows. ( b ) LEED pattern after formation of the second layer Pb taken using MCP-LEED optics (beam energy 24 eV). Full size image LEED was employed to determine the long-range order of the film. LEED taken from each of the Pb layers show fivefold patterns with spots at the same positions as the clean surface, as shown in Fig. 4b , which was recorded after formation of the second layer. This confirms that the Pb layers have quasicrystalline long-range order expected from the substrate. The LEED results are consistent with Fourier transforms of STM images, which exhibit tenfold symmetry with maxima located at τ scaling distances ( Fig. 3a , inset). The modulation in the autocorrelation of STM images extends up to maximum distances within the STM images without significant decrease in intensity ( Fig. 3a , inset). This also demonstrates an undiminished long-range order within the experimentally probed length scale. DFT calculations and comparison with STM To evaluate adsorption energies for Pb atoms on the i -Ag-In-Yb surface, we performed total energy calculations based on DFT using the VASP code [27] , [28] . Detail of the calculation are given in the Methods. The adsorption energy was calculated for different sites around the RTH cluster centre as a function of distance from the surface and optimal adsorption heights were identified. Four optimum heights were found. Three of them are at 0.5, 1.2 and 2.3 Å ( Fig. 5e,f ). The fourth one will be discussed later. The two-dimensional energy maps at 1.2 and 2.3 Å heights are plotted in Fig. 5a,b . These heights correspond to the height of the first and second Pb layers observed by STM microscopy. 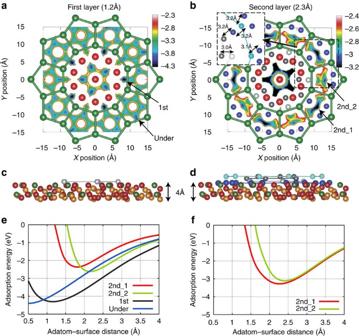Figure 5: Theoretical results for adsorption energies of the Pb layers. (a,b) Adsorption energy map for first and second layer Pb atoms around the RTH cluster centre, overlaid with atomic positions for the topmost substrate layer and Pb. Green spheres correspond to Yb, red to In, orange to Ag and other colours to Pb atoms. Inset shows the interatomic distances between adsorbed Pb atoms (see text). (c,d) Side view of atomic structure for the substrate and Pb film. (e,f) Adsorption energies for selected sites as a function of distance from the surface. Adsorption energy curves for 2nd_1 (red) and 2nd_2 (green) sites inewere calculated with the absence of the underlayer, and the same curves infare after the underlayer atoms are considered. The centre pentagonal sites ina(right) have the highest adsorption energy. We note that a repulsive interaction is expected between atoms adsorbed on centre pentagonal sites, shown inFig. 5b. Therefore, these sites may be occupied partially. However, adsorption behaviour at these sites is ambiguous because of lack of information of exact atomic structure at the centre of the RTH cluster. The adsorption energy is defined by, Figure 5: Theoretical results for adsorption energies of the Pb layers. ( a , b ) Adsorption energy map for first and second layer Pb atoms around the RTH cluster centre, overlaid with atomic positions for the topmost substrate layer and Pb. Green spheres correspond to Yb, red to In, orange to Ag and other colours to Pb atoms. Inset shows the interatomic distances between adsorbed Pb atoms (see text). ( c , d ) Side view of atomic structure for the substrate and Pb film. ( e , f ) Adsorption energies for selected sites as a function of distance from the surface. Adsorption energy curves for 2nd_1 (red) and 2nd_2 (green) sites in e were calculated with the absence of the underlayer, and the same curves in f are after the underlayer atoms are considered. The centre pentagonal sites in a (right) have the highest adsorption energy. We note that a repulsive interaction is expected between atoms adsorbed on centre pentagonal sites, shown in Fig. 5b . Therefore, these sites may be occupied partially. However, adsorption behaviour at these sites is ambiguous because of lack of information of exact atomic structure at the centre of the RTH cluster. Full size image thus, a larger negative value indicates a more stable site. In agreement with the STM observations, the most stable sites for the first layer are identified between the In and Yb rings, which make a pentagon around the RTH cluster centre. These sites are indicated as ‘1st’ in the figure. The expected structure of the first layer is represented by white spheres in the side view ( Fig. 5c,d ). After the formation of the first layer, Pb atoms are adsorbed at 0.5 and 0.6 Å above the surface. These underlayer sites are represented by blue spheres in the figure (refer to as Under). The energy curve for the adsorption sites at 0.5 Å is slightly different from the sites at 0.6 Å. We show the energy curve at 0.5 Å in Fig. 5e as a representative. After the underlayer sites are occupied, five deep minima (2nd_1) and the other shallow minima (2nd_2) are obtained at the centre of Yb pentagons surrounding the RTH cluster centre. These sites are at 2.3 Å from the surface and, thus, correspond to adsorption sites for the second layer. As the potential at the 2nd_1 site is slightly deeper than at the 2nd_2 site, a Pb pentagon forms first in the second layer rotated by 36 o compared with the pentagon in the first layer and larger by a factor of τ . This is observed by STM. After completion of the pentagon, the shallower 2nd_2 sites are occupied, forming a decagon, again consistent with the STM results. We also identify adsorption sites of two different types located near to the RTH cluster centre, which are represented by grey spheres in Fig. 5a,b . These sites appear slightly below the second layer and above the first layer. In addition, the calculation indicates the existence of stable adsorption sites above the second layer and around 2nd_1 and 2nd_2 sites. From the location and height distribution, we infer that these sites correspond to the intermediate layers identified by STM. The adsorption sites identified by STM and calculations are found to be identical to the atomic positions in the RTH cluster. The atoms of a given layer occupy sites of specific chemical species in the cluster. To demonstrate this, we present the atomic structure derived from the bulk model of i -Ag-In-Yb in Fig. 6 . The position and atomic density of the layers, which are formed by atoms of different shells of the RTH cluster, are given in Fig. 6a . The in-plane structure of the layers are shown in Fig. 6b–d . The atoms in the innermost tetrahedral shell are not shown, as their density is low. 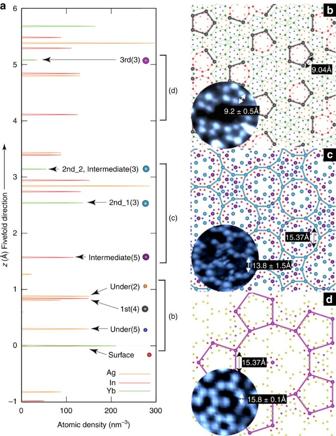Figure 6: Structure model of Pb layers. (a) The atomic density distribution ofi-Ag-In-Yb along the fivefold direction. The density is estimated in slabs of 0.01 Å thickness. The Yb rich at plane intersecting the centre of RTH cluster represents the topmost surface layer (z=0). Pb layers are formed at planes indicated by arrows. Thenth shell of the RTH cluster is indicated in parentheses. (b–d) The in-plane atomic structure in a slab marked ina(b, 0≤z≤0.90 Å;c, 1.53≤z≤3.15 Å;d, 5.04≤z≤5.40 Å). (b) The surface In and Yb atoms are plotted in small red and green spheres, respectively, and are connected by thin lines. In sites are plotted by large grey spheres and connected by thick lines. These sites are identical to the first layer Pb (see inset). (c) Yb (large blue) and In (large magenta) sites correspond to the second and intermediate Pb layers, respectively. (d) Yb (large purple) corresponds to the third layer Pb. Inset ofb–dis STM image of the first, second and third layer Pb, respectively. Figure 6: Structure model of Pb layers. ( a ) The atomic density distribution of i -Ag-In-Yb along the fivefold direction. The density is estimated in slabs of 0.01 Å thickness. The Yb rich at plane intersecting the centre of RTH cluster represents the topmost surface layer ( z =0). Pb layers are formed at planes indicated by arrows. The n th shell of the RTH cluster is indicated in parentheses. ( b – d ) The in-plane atomic structure in a slab marked in a ( b , 0≤ z ≤0.90 Å; c , 1.53≤ z ≤3.15 Å; d , 5.04≤ z ≤5.40 Å). ( b ) The surface In and Yb atoms are plotted in small red and green spheres, respectively, and are connected by thin lines. In sites are plotted by large grey spheres and connected by thick lines. These sites are identical to the first layer Pb (see inset). ( c ) Yb (large blue) and In (large magenta) sites correspond to the second and intermediate Pb layers, respectively. ( d ) Yb (large purple) corresponds to the third layer Pb. Inset of b – d is STM image of the first, second and third layer Pb, respectively. Full size image The surface plane is an Yb-rich layer intersecting the centre of the RTH clusters as described above. This plane is at z =0 in Fig. 6a . Arrows indicate the layers of atomic sites occupied by Pb. The n th shell of the RTH cluster is indicated in parentheses. Figure 6b is the in-plane structure for 0< z ≤0.9 Å. In sites of the fourth shell of the RTH cluster are plotted by large grey spheres. Most of these sites form a pentagon or a part of it, and the edge length of the pentagon agrees with that of the first-layer Pb pentagon obtained in experiment (9.2±0.5 Å). Figure 6c shows the in-plane structure of the range 1.53≤ z ≤3.15 Å, where the Yb sites (the third shell of the RTH cluster, blue spheres) form decagons. The edge length of the decagons matches again with that of observed second layer Pb (13.8±1.5 Å). We can also identify sites corresponding to the third layer Pb, which are presented in Fig. 6d . The edge length of the decagon in the model structure is also in agreement with that of the third layer Pb (15.8±1 Å). Similarly, the sites related to the under- and intermediate layers can also be derived from the model structure (shown in Fig. 6b,c , respectively). Although the lateral position of adsorption sites obtained in calculation agrees exactly with the bulk structure, the absolute heights of the layers differ slightly from the bulk values, probably because of the relaxation of the Pb layers due to the absence of the bulk structure in vacuum. The adlayer–adlayer interaction is crucial for stability of the Pb film. The calculation reveals that the second-layer Pb is significantly stable only if the underlayer is present. This is demonstrated in Fig. 5e,f , where we compare the adsorption energy curve for the second layer atoms with and without the existence of the underlayer. The adsorption energy of 2nd_1 and 2nd_2 sites increases by about 1 and 0.5 eV, respectively, after the formation of the underlayer. Similarly, the existence of the intermediate layer lowers the potential for the 2nd_1 site compared with the 2nd_2 site. This change in the potential landscape induced by the under- (and intermediate) layer explains the STM observations that the second-layer Pb pentagons are oriented by 36° with respect to the pentagons in the first layer, and they evolve to decagons with increasing Pb coverage. We also find another relationship that implies the importance of the order of adsorption between the first layer and underlayer. If the underlayer is formed before the first layer, the first layer Pb pentagons observed by STM cannot be produced by calculation. Furthermore, the interatomic distance between the adsorbed Pb atoms is short enough to conclude a strong interaction between the adatoms. These distances are shown in Fig. 5b (inset). The calculated values are shorter than the nearest neighbour distance in the fcc Pb (3.5 Å). We suggest that the shorter Pb–Pb distances are caused by attractive interactions with the substrate and perhaps also by underestimation of DFT. It is known that Pb is immiscible to Ag, but forms a solid solution with In, and forms several intermetallic compounds with Yb [29] . This suggests strong bonding for Pb–Yb and Pb–In. The top layer of the substrate in the present model consists of only In and Yb. This particular surface composition may be crucial for stabilizing the overlayer of Pb. Other elements such as Bi and Sb are expected to form strong bonds with Yb as characterized by the high melting temperature of intermetallic compounds of these elements [30] , [31] . Indeed, further STM measurements show both elements produce first and second layers on the same substrate, and preliminary DFT calculations also support the existence of stable pseudomorphic Bi and Sb layers. However, the detail of each Bi or Sb layer is different from that of Pb, possibly because the Bi–Bi or Sb–Sb distance in the bulk is slightly different from that of Pb. The details of the Bi and Sb results will be published elsewhere. The impact of our findings is fourfold. First, the proposed mechanism allows the prediction of other novel epitaxial material phases. Second, as all available bulk quasicrystals are associated with a complex chemistry, it has not been possible previously to separate the influence of quasicrystalline order and chemistry on the intriguing physical properties of quasicrystals. The single-element systems presented in this work exhibit quasicrystalline order with chemical simplicity and thus these can be used as model systems to study the impact of quasicrystalline order on physical properties, independent of chemical complexity. Third, the physical properties of a material are governed by atomic order. It will be of great interest to compare physical properties such as superconductivity between Pb in its natural periodic form and in the quasicrystalline allotrope. Fourth, element-specific experimental techniques can be employed to exclusively probe the quasicrystalline overlayer without a contribution from the underlying substrate. In conclusion, we have presented the first observations of three-dimensional growth of quasicrystalline thin film of a single element. The film is formed on the fivefold surface of the i -Ag-In-Yb quasicrystal. Employing the experimental techniques of STM, XPS, LEED and DFT calculations, we have determined the atomic structure of the film. The deposited Pb atoms occupy the atomic sites of the RTH cluster, the building block of the substrate, and thus grow in layers with different heights and different adsorption energies. The Pb–Pb atomic distance in the film is sufficiently short compared with the bulk Pb to indicate a strong adlayer–adlayer interaction, which stabilizes the layered structure. The discovery of such a template single-element quasicrystalline thin film presents several new and exciting opportunities for further investigation of the impact of quasicrystallinity on the chemical and physical properties of materials, such as the superconductivity of quasicrystalline Pb. Bulk structure of i -Ag-In-Yb The i -Ag-In-Yb quasicrystal is isostructural to the unique binary i -Cd-Yb phase [22] . The basic building block of this system is the RTH cluster, which consists of five successive atomic shells [23] . The atomic shells are a Cd rhombic triacontahedron (outermost), a Cd icosidodecahedron, a Yb icosahedron, a Cd dodecahedron and a Cd tetrahedron (innermost). The RTH clusters contain 93.8% of the total number of atoms in the crystal. The remaining atoms are contained in acute and obtuse rhombohedra, which provide linkages or ‘glue’ between the RTH units. Thin-film preparation Pb was deposited on the fivefold surface of i -Ag 42 In 42 Yb 16 at temperature of 300 K using an Omicron electron-beam evaporator with a constant flux. Before the deposition, the substrate was prepared and characterized as described in ref. 24 . The pressure during deposition remained almost the same as the base pressure. The Pb film was characterized by STM, LEED and XPS. STM measurements were performed at room temperature in constant current mode. XPS and STM experiments were performed in two chambers with different flux and geometry for Pb deposition. DFT calculations Calculations are done with projector-augmented-wave potentials [32] and the generalized gradient approximation [33] . To handle the aperiodic fivefold surface in the periodic calculation, the surface is approximated by a disc-shaped cluster with 4 Å thickness and 30 Å diameter. The atomic positions are extracted from a model for the isostructural Cd-Yb quasicrystal [23] . Chemical ordering of Ag and In is assumed according to the occupation probability deduced from an X-ray diffraction experiment for the cubic approximant as described in ref. 26 . The topmost layer is chosen to intersect the RTH cluster centre and is flat. With the chemical ordering assumed here, this flat layer consists of only In and Yb. This is consistent with the relaxation trend that Ag is more likely to intrude into the bulk [34] . Moreover, the innermost shell of the RTH cluster is a tetrahedron of In in the bulk, but the structure near the surface has not been determined yet. We assume here that there is a single In atom at the RTH cluster centre for the topmost layer. A convergence test for adsorption energies was performed by comparison with results for larger model-clusters with 30 Å diameter and 6 Å thickness, and 50 Å diameter and 4 Å thickness. In most cases, the maximum difference is less than 0.1 eV, and it is about 0.2 eV at worst. Relaxations of atomic positions and spin-polarization effects are not included in all calculations. How to cite this article: Sharma, H. R. et al . Templated three-dimensional growth of quasicrystalline lead. Nat. Commun. 4:2715 doi: 10.1038/ncomms3715 (2013).